Variation of a major facilitator superfamily gene contributes to differential cadmium accumulation between rice subspecies Cadmium (Cd) accumulation in rice grain poses a serious threat to human health. While several transport systems have been reported, the complexity of rice Cd transport and accumulation indicates the necessity of identifying additional genes, especially those that are responsible for Cd accumulation divergence between indica and japonica rice subspecies. Here, we show that a gene, OsCd1 , belonging to the major facilitator superfamily is involved in root Cd uptake and contributes to grain accumulation in rice. Natural variation in OsCd1 with a missense mutation Val449Asp is responsible for the divergence of rice grain Cd accumulation between indica and japonica . Near-isogenic line tests confirm that the indica variety carrying the japonica allele OsCd1 V449 can reduce the grain Cd accumulation. Thus, the japonica allele OsCd1 V449 may be useful for reducing grain Cd accumulation of indica rice cultivars through breeding. Cadmium (Cd) is a toxic heavy metal and can lead to Cd-related diseases such as renal tubular dysfunction and bone disease. Rice is a major component of diet for over half of the world's population. The accumulation of Cd is a serious threat to human being since it can be concentrated in body through the food chain [1] and the biological half-life is estimated to be nearly 30 years [2] . Molecular genetic tools have been urgently sought to develop low-Cd rice to reduce potential health risks. Generally, Cd is first absorbed from soil by roots, and then translocated into shoots, and accumulates into grains in final [3] . Transport systems, especially the genetic components locating on the membrane, play crucial roles in the Cd accumulation processes in rice. In root exodermis and endodermis, OsNramp1 [4] , [5] and OsNramp5 [6] , [7] , [8] , [9] , [10] , [11] , which locate on the plasma membrane, are transporters for Cd uptake. The heavy metal ATPase, OsHMA3 [12] , [13] , [14] , [15] , functions in vacuolar sequestration of Cd. In root stele, OsHMA2 [16] , [17] , [18] , an efflux-type metal transporter on the plasma membrane, is suggested to facilitate Cd loading into the xylem. CAL1, a defensin-like protein preferentially expressed in root exodermis and xylem parenchyma cells, drives long-distance Cd transport via xylem vessels [19] . And in shoot node, OsLCT1 [20] , [21] , a plasma membrane-localized efflux transporter, is responsible for Cd intervascular transfer. By over-expression of the functional OsHMA3 or the disruption of OsLCT1 and OsHMA2, the grain Cd content can be reduced to some extent, which gives a clue that rice grain Cd contents can be reduced through regulating transporters expression. However, the rice Cd transport mechanism is complex and grain Cd accumulation is a result of cooperative interactions among multiple cells and issues. It is, therefore, worthwhile to explore more genetic loci involving in Cd accumulation of rice grain. Rice varieties exhibit substantial genetic variation with respect to Cd accumulation ability [22] , [23] , [24] , which is a valuable resource for dissecting functional alleles and genetic improvement. OsHMA3 shows different Cd transport ability [13] and OsNRAMP1 expresses in a different level among two cultivars [4] . By using chromosome segment substitution lines (CSSLs) carrying segments of indica rice Kasalath in a background of the japonica rice Koshihikari, several CSSLs have significantly lower Cd concentrations than that of Koshihikari [25] . However, current understanding of the genetic basis of rice Cd accumulation diversity remains at the level of the identification of several quantitative trait loci (QTLs) [25] , [26] , [27] . The natural allelic variations responsible for rice varietal differences have not been fully explored and the genetic basis of grain Cd accumulation differences remains unknown. More recently, genome-wide association studies (GWAS) have been successfully used for identifying genes and alleles underlying several agronomic traits [28] , [29] , [30] , [31] , [32] , while the association study of rice grain Cd accumulation has not been attempted. Here, we show that a gene belonging to major facilitator superfamily, OsCd1 , is associated with divergence in rice grain Cd accumulation. OsCd1 locates at the plasma membrane of root and is involved in the grain Cd accumulation. Additionally, a single-nucleotide mutation, SNP22, diverges between indica and japonica and alters Cd transport ability of OsCd1 . Interestingly, the natural variation OsCd1 V449 in japonica , which is associated with a reduced Cd transport ability and decreased grain Cd accumulation, shows a potential value in low-Cd rice selection. OsCd1 is associated with grain cadmium accumulation in rice In this study, we combined data from GWAS, gene annotation in GO Slim database and the yeast assay to look for genes associated with rice grain Cd accumulation. A set of 127 rice cultivars including 41 japonica and 86 indica from mini-core collection of rice in China [33] and other wide-spread regions was used for GWAS of grain Cd concentration (Supplementary Fig. 1a, b ). After testing rice varieties with a Cd treatment assay, we found that indica varieties could be phenotypically distinguished from japonica varieties by their significantly higher grain Cd accumulation (Supplementary Fig. 1c and Supplementary Data 1 ). Using 3,291,150 single-nucleotide polymorphisms (SNPs) with a minor allele frequency (MAF) > 0.05 covering the whole rice genome, we performed GWAS to identify the genetic loci associating with grain Cd accumulation. Under the compressed general mixed linear model ( P < 1 × 10 −5 , MLM, threshold derived from 1000 permutation test) (Fig. 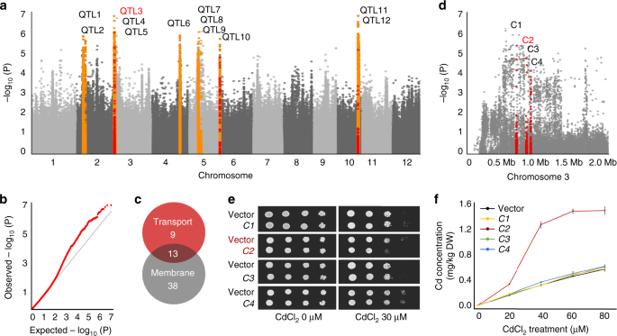Fig. 1 GWAS of the grain Cd accumulation.aManhattan plots for grain Cd accumulation in diverse population. The orange pots indicated the 12 QTLs were identified as significantly associated with grain Cd accumulation. The red dots indicated the 14 candidate genes associated both with transport and membrane in GO Slim annotation.bThe QQ plots for GWAS MLM model.cThe numbers of genes annotated with transport and membrane.dThe genome-wide association signals for grain Cd accumulation were shown in the region of 0–2 Mb on chromosome 3 (x-axis). The locations of four candidate genesC1(LOC_Os03g02150),C2(LOC_Os03g02380),C3(LOC_Os03g02390) andC4(LOC_Os03g02480) were indicated with red pot respectively.eDilution-series spot assays of yeast treated with and without 30 μM CdCl2.fCd accumulation in wild-type W303 (black) and W303 expressingC1(yellow),C2(red),C3(green) andC4(blue) treated with CdCl2for 24 h. Error bars indicate standard deviation. Data from the transgenic lines were designed with three replications and data points for all biological replicates are shown. Source data of Fig.1fare provided as a Source Data file 1a, b ), 12 QTLs were identified as significantly associated with grain Cd accumulation (Supplementary Table 1 ). According to the rice genome annotation project website (MSU-RGAP), 494 genes were annotated to be located in the candidate locus (Supplementary Data 2 ). To identify the membrane transporter conferring Cd accumulation in rice, we then performed the gene ontology (GO) Slim analysis to select candidate genes associated with the keyword membrane and transport for further research. Altogether, 13 candidate genes located on chromosome 2, 3, 4, 6, and 10 were found to be associated both with transport and membrane in GO Slim annotation (Fig. 1c and Supplementary Data 3 ). Four candidate genes were selected on QTL3 of chromosome 3, which explained ~20.7% of the phenotypic variation (Fig. 1d ), and transformed into S. cerevisiae to evaluate whether these candidate genes were involved in Cd transport. Fig. 1 GWAS of the grain Cd accumulation. a Manhattan plots for grain Cd accumulation in diverse population. The orange pots indicated the 12 QTLs were identified as significantly associated with grain Cd accumulation. The red dots indicated the 14 candidate genes associated both with transport and membrane in GO Slim annotation. b The QQ plots for GWAS MLM model. c The numbers of genes annotated with transport and membrane. d The genome-wide association signals for grain Cd accumulation were shown in the region of 0–2 Mb on chromosome 3 ( x -axis). The locations of four candidate genes C1 ( LOC_Os03g02150 ), C2 ( LOC_Os03g02380 ), C3 ( LOC_Os03g02390 ) and C4 ( LOC_Os03g0248 0) were indicated with red pot respectively. e Dilution-series spot assays of yeast treated with and without 30 μM CdCl 2 . f Cd accumulation in wild-type W303 (black) and W303 expressing C1 (yellow), C2 (red), C3 (green) and C4 (blue) treated with CdCl 2 for 24 h. Error bars indicate standard deviation. Data from the transgenic lines were designed with three replications and data points for all biological replicates are shown. Source data of Fig. 1f are provided as a Source Data file Full size image Spot assays were tested with and without 30 μM CdCl 2 and the growth rate was normalized by non-transgenic strains. As a result, only yeast transformed C2 ( LOC_Os03g02380 ; GenBank accessions AP014959.1) displayed sensitivity to Cd (Fig. 1e ). Under 24 h Cd exposure, expression of C2 enhanced Cd accumulation in a Cd dose-dependent manner while the other three showed no significant difference with the control (Fig. 1f ). These results indicated that C2 was the most likely candidate transporter gene in QTL3 and it was christened OsCd1 . 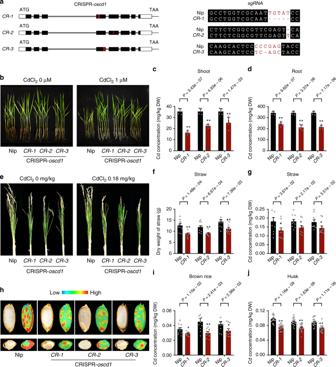Fig. 2 OsCd1contributes to the Cd uptake and grain accumulation in rice.aLeft: Schematic diagram of threeCRISPR-oscd1lines. Black rectangles represented exons ofOsCd1, red rectangle represented the exon of target sequence. Right: Sequences ofCRISPR-oscd1allelesCR-1,CR-2, andCR-3. sgRNA targets sequences were showed and deletions are indicated by red dashes.bGrowth of wild-type rice and threeCRISPR-oscd1lines after treating with and without 1 μM CdCl2for 20 days.c,d,g,i,jConcentration of Cd in the shoot (c), root (d), straw (g), brown rice (i) and husk (j).eGrowth of wild-type rice and threeCRISPR-oscd1lines after treated with and without 0.18 mg kg−1Cd in pot-test.fDry weight of straw wild-type rice and threeCRISPR-oscd1lines after treated with 0.18 mg kg−1Cd in pot-test.hSR-μXRF images of Cd distribution in the longitudinal (upper) and latitudinal (lower) sections of rice grain. The emission intensity of each pixel was normalized using the beam intensity as reference. TheCRISPR-oscd1lines were shown in red and the wild-type line was shown in black. Error bars indicate standard deviation in the hydroponic experiment and standard error of mean in pot-test. Statistical comparison was performed by one-sidet-test (*P< 0.05 and **P< 0.01). All data were compared with Nipponbare and designed with at least five replications and data points for all biological replicates are shown. Source data of Fig.2c, d, f, g, i, and jare provided as a Source Data file OsCd1 encoded a protein belonging to the MFS with 12 bilayer-spanning domains and the signature motif of MFS, G(93)slaD(97)kqG(100)rkR(103) [17] , located in the second cytoplasmic loop (Supplementary Figure 2a, b ). There were 149 MFS superfamily members in rice and several of them were predicted to transport various substrates (Supplementary Data 4 ). A phylogenetic tree was constructed for OsCd1 along with all the MFS proteins in rice (Supplementary Fig. 3 ). It was clearly shown that the proteins facilitating the same substrate transport shared a closer phylogenetic relationship, while OsCd1 clusters separately formed an unknown-function clade. Together with the yeast spot assay results, we deduced that OsCd1 may form a new-function clade in MFS involving in Cd transport. OsCd1 altered cadmium uptake and grain accumulation in rice Considering the possible function of OsCd1 in Cd transport, we transformed the CRISPR/Cas9 constructs in rice callus and regenerated the transgenic plants to investigate the role of OsCd1 in rice. Three Cas9-positive lines ( oscd1-cr1 , oscd1-cr2, and oscd1 - cr3 ), which had either an insertion or deletion of one or few bases at the target sequences and disrupted the Cd transport ability of OsCd1 (Supplementary Fig. 4 ), were selected for further research (Fig. 2a ). In vegetative growth stage, the growth without CdCl 2 treatment was not affected by the mutation of OsCd1 . After being treated with 1 μM CdCl 2 for 20 days, the CRISPR-oscd1 lines displayed a better growth (Fig. 2b ) and the Cd concentration both in root and shoot were much lower than that in the wild-type rice (Fig. 2c, d ). We then grew them in the field until ripening to investigate the physiological role of OsCd1 in grain Cd accumulation. At harvest, both the growth and the yield were affected by the disruption of OsCd1 (Fig. 2e ). The biomass of the straw (Fig. 2f ) and the filled spikelet were reduced in the mutant lines due to decreased fertility (Supplementary Fig. 5 ). As to the Cd concentration, the result showed that there was a decrease Cd accumulation in the straw of three CRISPR-oscd1 lines compared with the wild type (Fig. 2g ). The synchrotron radiation microscopic X-ray fluorescence (SR- μ XRF) scanning was further used to reveal the spatial disparity in the distribution of Cd throughout the grain in situ. As it is shown in Fig. 2h , Cd enriched both in the endosperm and aleurone layer, and its concentration was in a lower level in CRISPR-oscd1 lines than the wild type. Moreover, the Cd concentration was significantly decreased in brown rice and husk in three CRISPR-oscd1 lines, which was in well agreement with the SR- μ XRF results above (Fig. 2i, j ). The concentration of other micronutrients, including Zn, Mn, and Fe, were also detected in the CRISPR-oscd1 lines. Compared with the wild-type rice, no difference in the concentration of Zn and Fe was observed but Mn, which is important in photosynthetic oxygen evolution in chloroplasts of plants, displayed a significant decrease in the CRISPR-oscd1 lines (Supplementary Fig. 6 ). Fig. 2 OsCd1 contributes to the Cd uptake and grain accumulation in rice. a Left: Schematic diagram of three CRISPR-oscd1 lines. Black rectangles represented exons of OsCd1 , red rectangle represented the exon of target sequence. Right: Sequences of CRISPR-oscd1 alleles CR-1 , CR-2 , and CR-3 . sgRNA targets sequences were showed and deletions are indicated by red dashes. b Growth of wild-type rice and three CRISPR-oscd1 lines after treating with and without 1 μM CdCl 2 for 20 days. c , d , g , i , j Concentration of Cd in the shoot ( c ), root ( d ), straw ( g ), brown rice ( i ) and husk ( j ). e Growth of wild-type rice and three CRISPR-oscd1 lines after treated with and without 0.18 mg kg −1 Cd in pot-test. f Dry weight of straw wild-type rice and three CRISPR-oscd1 lines after treated with 0.18 mg kg −1 Cd in pot-test. h SR- μ XRF images of Cd distribution in the longitudinal (upper) and latitudinal (lower) sections of rice grain. The emission intensity of each pixel was normalized using the beam intensity as reference. The CRISPR-oscd1 lines were shown in red and the wild-type line was shown in black. Error bars indicate standard deviation in the hydroponic experiment and standard error of mean in pot-test. Statistical comparison was performed by one-side t -test (* P < 0.05 and ** P < 0.01). All data were compared with Nipponbare and designed with at least five replications and data points for all biological replicates are shown. Source data of Fig. 2c, d, f, g, i, and j are provided as a Source Data file Full size image To determine the expression profile of OsCd1 in rice, we analyzed the expression level from root and shoot at vegetative growth stage in rice via qPCR. The results showed that OsCd1 was mainly detected in roots, which was consistent with the GUS histochemical assay, and not induced by CdCl 2 (Fig. 3a ). The cell-specific expression of OsCd1 in rice root tissues was further analyzed using the GUS and GFP reporter fused to the OsCd1 promoter. The promoter activity of OsCd1 was mainly detected in the root exodermis, parenchyma in cortex, endodermis and stele cells (Fig. 3b–d and Supplementary Fig. 7 ). We then constructed the GFP fusion protein to examine the subcellular location of OsCd1 in rice. The green fluorescence was mainly localized in the cytosol and nucleus of cells expressing GFP alone while the OsCd1 fused with GFP was only observed at the periphery of the cells both in root cells and protoplast. The merged images of GFP and plasma membrane marker FM4-64 further confirmed the plasma membrane subcellular localization of OsCd1 (Fig. 3e, f ). Together with the CRISPR-oscd1 results, it is suggested that the OsCd1 , which was a plasma membrane protein in root, may be involved in Cd uptake and contributed to grain Cd accumulation in rice. Fig. 3 Expression pattern of OsCd1 in rice. a Tissue-dependent expression of OsCd1 at vegetative stage. Left: GUS histochemical assay of the transgenic plant with the GUS reporter driven by the OsCd1 promoter. Right: the expression level of OsCd1 in root and shoot with and without 1 μM CdCl 2 treatment via qPCR. Bars = 2 mm. b Tissue-specific localization of OsCd1 in the root of rice using the GUS reporter driven by the OsCd1 promoter. Bars = 0.5 mm. c Tissue-specific localization of OsCd1 in the root of rice using the GFP driven by the OsCd1 promoter in cross frozen sections. Nip, negative control; Ubi::GFP, positive control. Bars = 10 μm. d The GFP transcriptional level shown by RT-PCR. Upper, GFP ; Down, Actin . e Subcellular location of OsCd1 in the root of rice observed by confocal laser scanning microscopy. The GFP fluorescence, fluorescence of FM4-64 and overlay of FM4-64 and pMDC45 -GFP (left), OsCd1 -GFP (right) were shown, respectively. Bars = 20 μm. f Subcellular location of OsCd1 in root protoplasts. Bars = 10 μm. Source data of Fig. 3a and d are provided as a Source Data file Full size image SNP22 altered the cadmium transport ability of OsCd1 The full-length sequences of 127 rice cultivars were used to investigate functional allelic variations in OsCd1 locus. A total of 24 SNPs were identified in the OsCd1 genomic region: 3 SNPs in the 5′UTR, 3 SNPs in the exon, 17 SNPs in the intron and 1 SNP in the 3′UTR, respectively (Supplementary Data 5 ). In specific, only the SNP22 (g. 846037 T>A), a missense mutation in eighth exon, resulted in a negative amino acid valine corresponding to a neutral one aspartic (a p. Val449Asp substitution) (Fig. 4a ). OsCd1 was a typical MFS protein with 12 transmembrane a-helices. Additionally, there were three extra intracellular helical domains (ICHs) on the intracellular side, one at the C terminus (ICH1) and the other two (ICH2 and ICH3) locating between the amino- and C-terminal TM bundles. The amino acid substitution V449D located on the C-terminal and around the ICH1 from the cytoplasmic face of the plasma membrane (Fig. 4b ). Fig. 4 Functionally important amino acids in OsCd1 . a Schematic diagram of gene structure and SNPs in OsCd1 . b Predicted three-dimensional structural model of OsCd1. The structures of O s C d 1 D449 (red) were viewed parallel (left one) and perpendicular (right one) to the membrane, respectively, and so for OsCd1 V449 (gray). Residue Asp449 in OsCd1 D449 (red) and Val449 in OsCd1 V449 (gray) were labeled at the cytoplasmic end respectively. ICH indicated intracellular helix. All structure figures were prepared with PyMol. c The grain Cd distribution of each genotype of OsCd1 among rice natural variations group treated with 0.18 mg kg −1 in pot-test; n denoted the number of genotypes belonging to each group. In each box plot, the bold horizontal line indicates the median, the edges of the box represent the first and third quartiles, and whiskers extend to span a 1.5 interquartile range from the edges. d Cd accumulation in W303 expressing OsCd1 D449 (red) and OsCd1 V449 (black) yeast treated with 20, 40, 60, 80 μM CdCl 2 for 24 h. Data from the transgenic lines were designed with three replications. e SR- μ XRF images of Cd distribution of ZH11, OE-OsCd1 V449 , and OE-OsCd1 D449 lines in the rice grain. The emission intensity of each pixel was normalized using the beam intensity as reference. f Concentration of Cd in the brown rice of ZH11 (gray), OE-OsCd1 V449 (black) and OE-OsCd1 D449 (red) lines treated with 1.8 mg kg −1 in the field. Error bars indicate standard deviation. Statistical comparison was performed by one-side t -test (* P < 0.05 and ** P < 0.01). Data from the transgenic lines were designed with ten replications and data points for all biological replicates are shown. Source data of Fig. 4c, d and f are provided as a Source Data file Full size image To find the haplotype between SNP22 with rice grain Cd accumulation, we then conducted the haplotype analysis for SNP22 and grain Cd accumulation in 127 rice cultivars. The results showed that the OsCd1 can be classified into two genotypes based on the SNP22: OsCd1 D449 with the A on SNP22 ( n = 82) and OsCd1 V449 with the T on SNP22 ( n = 34). Statistically, lines with OsCd1 D449 have an ~2-folds grain Cd concentration compared to those with OsCd1 V449 ( P = 6.68 × 10 −8 ) (Fig. 4c ) but with no obvious difference in expression levels and subcellular location (Supplementary Fig. 8 and 9 ). We further analyzed the Cd concentration in OsCd1 V449 and OsCd1 D449 transgenic yeast strains to investigate if the variation caused by SNP22 might alter the Cd transport ability of OsCd1 . As shown in Fig. 4d and Supplementary Fig. 10 , OsCd1 D449 resulted in a higher Cd concentration compared to OsCd1 V449 under Cd treatment. Meanwhile, the expression level showed that there was no significant difference between the OsCd1 V449 and OsCd1 D449 transgenic lines with or without Cd treatment (Supplementary Fig. 11 ). To determine whether SNP22 led to alteration of grain Cd accumulation in rice, we generated transgenic lines by overexpressing the OsCd1 V449 and OsCd1 D449 in a ZH11 background. Both the OE-OsCd1 V449 and OE-OsCd1 D449 transgenic lines accumulated more Cd compared to ZH11. In addition, the transgenic lines of OE-OsCd1 V449 showed a significantly less Cd accumulation ability in rice grain than OE-OsCd1 D449 (Fig. 4e, f ). We then conducted the functional complementation assay by crossing both NILs with the OsCd1 D449 and OsCd1 V449 to the CRISPR-oscd1 knockout lines and treated the F1s with 1.8 mg kg −1 Cd in the field. At harvest, we measured the Cd concentration in the grain and it was observed that a higher level in F1s with OsCd1 D449 than that of F1s with OsCd1 V449 (Supplementary Figure 12 ). Together with the results in yeast systems, we concluded that the SNP22, resulting in a change of encoded amino acid, altered the Cd transport ability of OsCd1 . OsCd1 V449 introgression reduced grain cadmium accumulation Considering that OsCd1 V449 exhibits lower Cd transport ability than that of OsCd1 D449 , we generated near-isogenic line (NIL) by the introgression OsCd1 V449 of Nipponbare ( japonica ) into the background of 9311 ( indica with OsCd1 D449 genotype) for further research (Supplementary Figs. 13a and b ). The effect of the allele makeup at OsCd1 on grain Cd accumulation was firstly investigated in 0.18 mg kg −1 treated pot-grown rice at greenhouse. As it is shown in Supplementary Fig. 13c and d , 9311 displayed higher Cd concentration in rice grain than the female parent Nipponbare lines. With the introgression of OsCd1 V449 , the Cd accumulation of NIL was significantly reduced both in brown rice and husk compared with the 9311 backgrounds with no apparent difference in growth (Fig. 5a–c ). Fig. 5 OsCd1 V449 introgression reduces grain Cd accumulation. a Growth of 9311 and NIL after treated with or without 0.18 mg kg −1 Cd in pot-test. b , c Concentration of Cd in the brown rice and husk. Error bars indicate standard error of mean; statistical analysis was inspected using one-side paired t -test (* P < 0.05 and ** P < 0.01). d Growth and grain morphologies of 9311 and NIL after treated with 1.8 mg kg −1 Cd in the field. e Plant height of 9311 and NIL. f Actual yield per plot of 9311 and NIL. g SR- μ XRF images of Cd, Mn, Zn, Fe distribution in the longitudinal sections of rice grain. The emission intensity of each pixel was normalized using the beam intensity as reference. h – o Concentrations of Cd, Mn, Zn, Fe in the brown rice ( h , j – l ) and husk ( i , m – o ). 9311 were shown in red and the NIL was shown in black. In each box plot, the bold horizontal line indicates the median, the edges of the box represent the first and third quartiles, and whiskers extend to span a 1.5 interquartile range from the edges. Error bars indicate standard deviation. Statistical analysis was inspected using one-side t -test (* P < 0.05 and ** P < 0.01). All data were compared with 9311 and designed with at least five replications and data points for all biological replicates are shown. Source data of Fig. 5b, c, e, f, and h–o are provided as a Source Data file Full size image To evaluate the effect of OsCd1 V449 allele in vitro, we selected the Cd-polluted fields at Changsha (Hunan Province, China, E112°, N28°) [18] with 1.8 mg kg −1 Cd to perform the field trial. According to the newly published National Standard of the People’s Republic of China: Soil environment quality Risk control standard of soil contamination of agricultural land (GB15618-2018), the risk intervention values for Cd is set to 1.5 mg kg −1 (pH ≤ 5.5) or 2.0 mg kg −1 (5.5 < pH ≤ 6.5) [34] . The experimental level of Cd used in this filed is representative of a general situation of Cd-contaminated paddy fields in China. At harvest, there was no apparent difference in plant growth between the NIL and 9311. Moreover, the filled spikelet and actual yield per plot were also not affected by the introgression of OsCd1 V449 (Fig. 5d–f ). Notably, the grain Cd concentration was detected to be reduced in NIL (Fig. 5h, i ). According to the SR- μ XRF results, the Cd distribution in whole grain of NIL, especially the edible part endosperm, were significantly less than that in 9311 (Fig. 5g ). For other micronutrients, except for a slightly decrease of Mn, no obvious change in the concentration of Zn and Fe was observed between 9311 and NIL (Fig. 5g, j–o ). Additionally, when OsCd1 V449 was introduced into GUICHAO-2, another indica cultivar widely cultivated in south China, the grain Cd accumulation was also substantially decreased (Supplementary Fig. 14 ). These results demonstrated that the allelic effect of OsCd1 V449 contributed to the reduction of Cd in rice and, furthermore, may have a widely potential application value in rice genetic improvement. OsCd1 diverged between indica and japonica subspecies Interestingly, it was also observed that the OsCd1 in most of the indica accessions was with OsCd1 D449 (A at SNP22 site) and that in most of the japonica accessions was with the OsCd1 V449 (T at SNP22 site) (Supplementary Table 2 ). In special, the grain Cd accumulation level was significantly lower in the indica cultivars with OsCd1 V449 than that of OsCd1 D449 (Supplementary Fig. 15 ), indicating that the Cd accumulation of indica cultivars with OsCd1 V449 also fitted the regular pattern for japonica rice. To explore the phylogenetic relationship of this allele, we then used whole-genome sequencing data for a large panel of accessions [35] containing 446 O. rufipogon accessions and 950 O. sativa varieties to determine the ancestral states of the SNP22 in OsCd1 . Phylogenetic analysis using the 950 cultivar rice accessions showed that all the japonica accessions have nucleotide T (genotype OsCd1 V449 ) at SNP22 while 99% of the indica accessions have nucleotide A (genotype OsCd1 D449 ). Moreover, both the nucleotide A and T in SNP22 retained in its ancestor O. rufipogon (Fig. 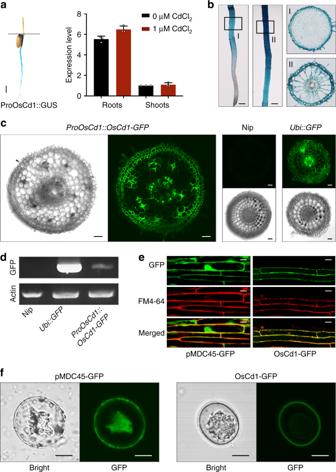Fig. 3 Expression pattern ofOsCd1in rice.aTissue-dependent expression ofOsCd1at vegetative stage. Left: GUS histochemical assay of the transgenic plant with the GUS reporter driven by theOsCd1promoter. Right: the expression level ofOsCd1in root and shoot with and without 1 μM CdCl2treatment via qPCR. Bars = 2 mm.bTissue-specific localization ofOsCd1in the root of rice using the GUS reporter driven by theOsCd1promoter. Bars = 0.5 mm.cTissue-specific localization ofOsCd1in the root of rice using the GFP driven by theOsCd1promoter in cross frozen sections. Nip, negative control; Ubi::GFP, positive control. Bars = 10 μm.dThe GFP transcriptional level shown by RT-PCR. Upper,GFP; Down,Actin.eSubcellular location ofOsCd1in the root of rice observed by confocal laser scanning microscopy. The GFP fluorescence, fluorescence of FM4-64 and overlay of FM4-64 andpMDC45-GFP (left),OsCd1-GFP (right) were shown, respectively. Bars = 20 μm.fSubcellular location ofOsCd1in root protoplasts. Bars = 10 μm. Source data of Fig.3a and dare provided as a Source Data file 6a , Supplementary Table 3 ). Fig. 6 Genotypes and phylogenetic analysis of OsCd1 . a The spectrum of allele frequencies at the causal polymorphisms of OsCd1 in O. rufipogon (Or-I, Or-II and Or-III) and O. sativa ( japonica and indica ). b Phylogenetic tree of the full population calculated from the SNPs of OsCd1 in O. sativa ( indica and japonica subspecies, up) and O. rufipogon (Or-I, Or-II and Or-III, down). c Phylogenetic tree of the full population calculated from the SNPs of OsCd1 in O. rufipogon (outer ring) and O. sativa (inner ring). d Illustration of genetic diversity and population differentiation in O. rufipogon and O. sativa . The F st values between the groups were indicated. ind, indica ; jap, japonica . Or-I, Or-II and Or-III are colored in pink, light blue and gray respectively; indica and japonica subspecies are in red and black, respectively Full size image Based on phylogenetic tree and PCA analysis, it was demonstrated that OsCd1 diverged between indica and japonica subspecies in cultivated rice and between subgroup Or-I and Or-III in wild rice (Fig. 6b ). Further analysis revealed that OsCd1 in indica was descended from O. rufipogon Or-I, which mainly distributes in South and Southeast Asia, while that in japonica was from Or-III, which mainly distributes in China [19] (Fig. 6c and Supplementary Figure 16 ). The level of population differentiation ( F st ) was estimated to be 0.06 in O. rufipogon and increased to 0.11 in O. sativa during domestication (Fig. 6d ). No significant Tajima’s D values were observed for japonica (Tajima’s D -1.16) and indica (Tajima’s D -1.32) cultivars, indicating that the divergence of OsCd1 between indica and japonica did not subject to selection and derived from the divergence of their progenitor gene pools hundreds of thousands of years ago. Reducing rice grain Cd accumulation is an important task for decreasing risks to human health. Rice absorbed Cd from soil by roots and finally transferred then into grain via transport systems. Thus, identifying the genetic components underlying Cd transport is of great importance to reduce Cd accumulation in rice grain. More recently, GWAS has been successfully used for dissecting loci in several important agronomic traits [28] , [29] , [30] , [31] , [32] and was a promising strategy for finding genetic variants underlying the grain Cd accumulation in rice. In this study, we analyzed the rice grain Cd contention in 127 varieties and performed GWAS to dissect the valuable genetic components underlying rice grain Cd accumulation (Fig. 1a–d ). As a result, QTL3, which showed the greatest contribution to the phenotypic variation, was selected for further research. Totally, 126 predicted genes with the annotation, such as transporter and transcription factor, were identified and may be the possible functional components in QTL3 (Supplementary Data 2 ). Using a composite bioinformatics tool-box method, OsCd1 , which belongs to the major facilitator superfamily (MFS), was detected to be associated with rice grain Cd accumulation on the whole-genome scale and confirmed to mediate Cd influx into cell in yeast system (Fig. 1e, f ). MFS is the largest group of secondary active membrane transporters, and its members transport a diverse range of substrates [36] . Recently, MFS proteins were reported to be functioned as transporters of some metal elements such as Arabidopsis zinc (Zn) transporter ZIF1 [37] and Arabidopsis cesium (Cs) and potassium (K) transporter ZIFL2 [38] , whereas the role of MFS proteins in Cd transport was still not clear. Here, we characterized the MFS protein OsCd1 as a possible Cd transporter gene in rice and the disruption of OsCd1 resulted in a decrease of Cd accumulation in root, shoot, and grain (Fig. 2 ). Furthermore, subcellular and tissue localization showed that OsCd1 was a plasma membrane protein and mainly expressed in the root exodermis, cortex, endodermis, and stele cells tissue (Fig. 3 ). We could then speculate that OsCd1 may mediate the Cd uptake in rice root and, ultimately, contribute to grain Cd accumulation. Together with the results in transgenic yeast and CRISPR-oscd1 lines, we thus deduced that OsCd1 may form a new-function clade in MFS involving in Cd transport. The exact role of OsCd1 in Cd accumulation, however, needed to be further explored. The identification of OsCd1 enables us to reduce Cd accumulation in rice grain by transgenic techniques. However, the disruption of OsCd1 is likely to result in a decrease of growth at harvest (Fig. 2e and Supplementary Fig. 5 ). As it was reported previously, OsCd1 ( ASL ) shares 93.2% similarity to the gene ASY , which regulates early shoot development in rice. The absent of ASY showed various shoot abnormalities at the early vegetative stage. OsCd1 ( ASL ) exists in the rice genome and is supposed to have redundant functions. For the reason that the OsCd1 ( ASL ) expression level increased at later stages, it was speculated that OsCd1 ( ASL ) may be involved in the shoot development of later stages [39] . In addition, it was also observed that OsCd1 influences the Mn accumulation while the exact mechanism needs to be further investigated (Supplementary Fig. 6 ). Mn is a required trace mineral for all known living organisms and functions as cofactors for a large variety of enzymes with many functions [40] , [41] and the disruption of OsCd1 was likely to influence the rice growth at harvest. Considering the fact that the disruption of OsCd1 has a negative impact on plant growth and reduces yield at harvest, it is thus not an optimal strategy to establish low-Cd rice by simply knocking out OsCd1 , while selection of superior alleles of OsCd1 may be a more effective strategy for genetic improvement of rice. We then conducted research to excavate natural variation allele in OsCd1 . Based on the sequences, we identified a nonsynonymous mutation (SNP22), locating at the ICH1 of C-terminal (Fig. 4a, b ), could cause a charged amino acid D449 substituting to an uncharged one V449. Typically, MFS protein possesses 12 transmembrane a-helices with both their N- and C-terminal located in the cytoplasm [42] , [43] , [44] , [45] , [46] . During the transport reaction cycle, some amino acids on N- and C-terminal form hydrogen bonds with the substrate and translocate the substrate via the “rocker-switch” mechanism [42] , [47] , [48] . N- and C-terminal, especially the charged or polar residues in the ICH domain, are likely to have a critical role to close the transporter on the intracellular side during the alternating access cycle [49] . When the V449 was substituted to D449 in SNP22, the polarity change caused a relatively stronger Cd transport ability in OsCd1 D449 compared with OsCd1 V449 (Fig. 4d ). The yeast essay, together with the complementary experiments with over-expression promoter indicated that the Cd transport ability varied in two alleles (Fig. 4e, f ). Considering native promoter, which is a better strategy for functional complementation, was not used, we thus crossed the alternative alleles to the CRISPR-oscd1 lines and the Cd transport ability variation was furtherly confirmed (Supplementary Fig. 12 ). The difference in Cd transport ability, finally, endowed the OsCd1 D449 rice cultivars with a higher grain Cd accumulation ability than the cultivars with OsCd1 V449 (Fig. 4c ). In addition, no tissue expression level and subcellular location differences were observed between the OsCd1 V449 and OsCd1 D449 (Supplementary Figs. 8 and 9 ). We thus regarded SNP22 in OsCd1 as a critical allele contributing to the divergence in rice grain Cd accumulation and tried to apply the functional allele OsCd1 V449 for marker-assisted breeding. Two rice cultivars, 9311 and GUICHAO-2, which showed a relatively higher grain Cd content compared with Nipponbare and Guihuahuang, were selected as the background of NIL. When the OsCd1 V449 allele was introduced into them, lower grain Cd accumulation NILs were obtained (Fig. 5b, c, h, i and Supplementary Fig. 14 ). Meanwhile, it is noteworthy that, different from CRISPR-oscd1 lines, which resulted in a complete loss of gene function, the NIL with lower grain Cd accumulation has no apparent difference in plant growth and spikelet fertility compared with 9311, though the Mn accumulation in NIL was slightly decreased (Fig. 5d–f and Supplementary Fig. 14 ). This suggests OsCd1 V449 a great potential application in low-Cd rice cultivation. Phylogenetic and population genetic analyses demonstrated the natural variation in OsCd1 diverged between indica and japonica subspecies: the japonica accessions with genotype OsCd1 V449 displayed a relatively lower Cd accumulation in rice grain than the indica accessions with genotype OsCd1 D449 (Fig. 6 ). This was different with OsNramp5 , a major Cd transporter in rice. In OsNramp5 , the frequency of the two missense variation SNPs in OsNramp5 showed almost no difference in indica and japonica , indicating it contributed little to the Cd divergency between indica and japonica rice (Supplementary Fig. 17 ). In Asia, the cultivated rice is mainly classified into indica and japonica subspecies. Indica cultivars, which are the major food and widely grown in the South and Southeast Asia, generally exhibit higher grain Cd accumulation than japonica cultivars [50] , [51] (Supplementary Fig. 1c ). Since Cd is one of the most serious soil heavy metal pollutant in these regions [52] , [53] , the ingestion of indica rice grain brings an unneglectable risk of Cd to people living there. In the previous study, three osnramp5-1 rice mutants were developed by carbon ion-beam irradiation strategy for marker-assisted selection of low-Cd cultivars [11] . However, the parent of these three rice mutants is Koshihikari, which is the main cultivar in Japan but not in China and other Southeast Asian countries. OsCd1 V449 exists in most of the japonica cultivars which makes it a wider parent selection range in low-Cd cultivar breeding. By integrating the low-Cd allele OsCd1 V449 into indica cultivars, the grain Cd accumulation had been successfully reduced on the Cd-contaminated paddy fields in Hunan province, where is considered as a typical Cd-contaminated area in China and has suffered from Cd contamination for many years. This finding, along with the function characterizing of natural variation of OsCd1 , emphasizes the potential application value of OsCd1 V449 in low-Cd rice cultivation, especially in indica cultivars. GWAS analysis and gene annotation A diverse worldwide collection of 127 O. sativa accessions including both landraces and elite varieties was obtained from a core/mini-core collection of Oryza sativa L. for GWAS analysis [33] . Each accession was germinated and planted in cultivation pot treated with 1.8 mg kg −1 Cd (Beijing, China; 39.9°N, 116.3°E). The grain was collected after harvest to test the Cd concentration of each genotype. In total, we used 3,291,150 SNPs with a minor allele frequency of >0.05 to carry out GWAS. Association analysis using a mix model was performed with the GAPIT software package. The top three principal components were used as fixed effects, and the matrix of genetic similarity based on simple SNP matching coefficients was used to model the variance-covariance matrix of the random effect. The analyses were performed in GAPIT and the parameters for each trait were optimized automatically. Permutation tests were used to help define the genome-wide significant P -value threshold [54] . For all the examined traits, we reshuffled the original phenotype data, and then performed association analysis using GAPIT with the same parameters. There ought to be no real associations between the SNPs and the simulated phenotypes, so all the SNPs passing the permutation threshold should be positives. After conducting 1000 permutation analyses, we clearly found that the permutation threshold varied across genomic region and some of the association signals even passing the significant cutoff 10 −5 . Thus, we adopted a threshold P = 10 −5 at genome-wide level. For QTL and gene annotation, we firstly selected the SNP signal that passing the threshold at P = 10 −5 , to check if the distance to the adjacent SNP was less than 170 kb [32] . We then merged it into the same QTL, all the genes locating in the QTL region were predicted by the Rice Genome Annotation Project (MSU-RGAP, Nipponbare version 6.1, http://rice.plantbiology.msu.edu/cgi-bin/gbrowse/rice/ ) and annotated by gene ontology (GO) Slim annotation with the keyword membrane and transport. 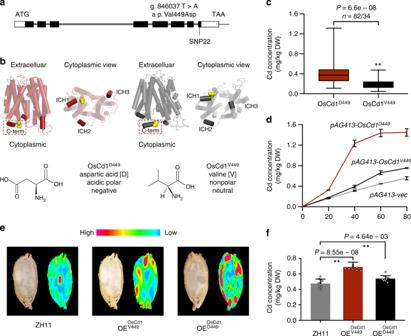Fig. 4 Functionally important amino acids inOsCd1.aSchematic diagram of gene structure and SNPs inOsCd1.bPredicted three-dimensional structural model of OsCd1. The structures ofOsCd1D449(red) were viewed parallel (left one) and perpendicular (right one) to the membrane, respectively, and so forOsCd1V449(gray). Residue Asp449 inOsCd1D449(red) and Val449 inOsCd1V449(gray) were labeled at the cytoplasmic end respectively. ICH indicated intracellular helix. All structure figures were prepared with PyMol.cThe grain Cd distribution of each genotype ofOsCd1among rice natural variations group treated with 0.18 mg kg−1in pot-test;ndenoted the number of genotypes belonging to each group. In each box plot, the bold horizontal line indicates the median, the edges of the box represent the first and third quartiles, and whiskers extend to span a 1.5 interquartile range from the edges.dCd accumulation in W303 expressingOsCd1D449(red) andOsCd1V449(black) yeast treated with 20, 40, 60, 80 μM CdCl2for 24 h. Data from the transgenic lines were designed with three replications.eSR-μXRF images of Cd distribution of ZH11,OE-OsCd1V449, andOE-OsCd1D449lines in the rice grain. The emission intensity of each pixel was normalized using the beam intensity as reference.fConcentration of Cd in the brown rice of ZH11 (gray),OE-OsCd1V449(black) andOE-OsCd1D449(red) lines treated with 1.8 mg kg−1in the field. Error bars indicate standard deviation. Statistical comparison was performed by one-sidet-test (*P< 0.05 and **P< 0.01). Data from the transgenic lines were designed with ten replications and data points for all biological replicates are shown. Source data of Fig.4c, d and fare provided as a Source Data file Primers The sequences for all primers used in this study are listed in Supplementary Table 4 . Cadmium and manganese transport activities assay in yeast RNA was extracted from CRISPR-oscd1 , 9311 and Nipponbare accessions. For candidate gene selection assay, the coding sequence of C1 , C2 , C3 , and C4 was amplified from 9311 cDNA. The haplotypes OsCd1 V449 and OsCd1 D449 were amplified from 9311 and Nipponbare cDNA, respectively. The oscd1-CR1 , oscd1-CR2 and oscd1-CR3 were amplified from CRISPR-oscd1 , respectively. The sequences were then cloned into pAG413GAL vector to construct yeast expression vector. The constructed vectors along with the empty vector pAG413GAL were transformed into the wild-type Saccharomyces cerevisiae W303 ( MATa his3-1 met15-0 trp1-1 ura3 , Laboratory preservation), Δycf1 (MATa ura3 leu2 his3-1 met15-0 YDR135c::kanMX4 , Laboratory preservation) and Δsmf1 (MATa his3-1 leu2 met15-0 ura3 YOL122c::kanMX4 , Chen Caiyan’s Laboratory preservation). Polyethylene glycol (PEG)/LiAc-based method was used for preparing and transforming competent yeast cells [55] . Yeast cells were grown at 30 °C in YPAD medium and then treated with 100 mM LiAc to make yeast competent cells. The mixture of ~200 ng μl −1 plasmid, 240 μl PEG solutions, 26 μl 1 M LiAc and 10 μl Carrier DNA were added into the yeast competent cells and incubated at 30 °C for 30 min. Then the mixture was heat shocked at 42 °C for 20 min. Yeast transformants were cultured in synthetic defined (SD) medium without histidine at 30 °C for 48 h. For plate growth tests, yeast transformants were diluted to an OD 600 of 1.0, 0.1, 0.01, and 0.001 step by step with sterile water. Then the yeast transformants were spotted on SD-His plates (with 2% (w v −1 ) galactose/glucose) with or without 30 μM CdCl 2 or 5 mM EGTA, respectively. The yeast carrying empty vector was used as control. Plates were incubated for 2–3 d at 30 °C for phenotype observation. All the assays were performed at least three times. For the Cd and Mn concentration determination, the yeast transformants were cultured overnight with liquid SD medium (with 2% galactose) to OD 600 = 1 with 200 rpm at 30 °C. Then the yeast transformants were treated with 20, 30, 40, 60, 80 μM CdCl 2 for 24 h or 5 mM EGTA for 48 h, respectively. The yeast strain carrying empty vector was used as control. All the yeast samples were collected and washed with sterile water for three times. Then all the samples were dried at 80 °C in an oven for further Cd and Mn concentration determination. All the assays were performed at least three times. 3D structure modeling and protein structure analysis The OsCd1 sequence was analyzed by Phyre2 [56] and secondary structure was displayed using TMRPres2D [57] to determine the position of the transmembrane helices. Three-dimensional model of OsCd1 V449 and OsCd1 D449 were constructed using the Phyre2 and MODELLER software [58] . Three high-resolution protein structures GlpT (PDB entry 1pw4), YajR (PDB entry 3wdo), and POT (PDB entry 4iky) were used as templates simultaneously in the comparative modeling procedure. Three-dimensional models were visualized within PyMOL [59] . Phylogenetic reconstruction of OsCd1 In total 149 protein sequence of MFS members from rice were obtained from Transport Database ( http://www.membranetransport.org/transportDB2/index.html ). Multiple-sequence alignment was optimized by MUSCLE. The phylogeny of OsCd1 in the MFS was constructed by MEGA7 [60] using the neighbor-joining method with No. of differences model, pairwise deletion for missing data and 1000 bootstrap pseudoreplicates. The software EvolView [61] was used for visualizing the phylogenetic trees. CRISPR-oscd1 mutant lines and function complementary essay The sgRNA-Cas9 and pUN1301-OsCd1 plant expression vectors were constructed [62] . 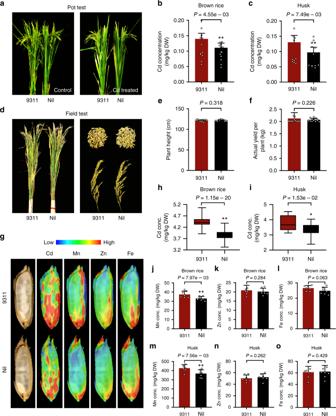Fig. 5 OsCd1V449introgression reduces grain Cd accumulation.aGrowth of 9311 and NIL after treated with or without 0.18 mg kg−1Cd in pot-test.b,cConcentration of Cd in the brown rice and husk. Error bars indicate standard error of mean; statistical analysis was inspected using one-side pairedt-test (*P< 0.05 and **P< 0.01).dGrowth and grain morphologies of 9311 and NIL after treated with 1.8 mg kg−1Cd in the field.ePlant height of 9311 and NIL.fActual yield per plot of 9311 and NIL.gSR-μXRF images of Cd, Mn, Zn, Fe distribution in the longitudinal sections of rice grain. The emission intensity of each pixel was normalized using the beam intensity as reference.h–oConcentrations of Cd, Mn, Zn, Fe in the brown rice (h,j–l) and husk (i,m–o). 9311 were shown in red and the NIL was shown in black. In each box plot, the bold horizontal line indicates the median, the edges of the box represent the first and third quartiles, and whiskers extend to span a 1.5 interquartile range from the edges. Error bars indicate standard deviation. Statistical analysis was inspected using one-sidet-test (*P< 0.05 and **P< 0.01). All data were compared with 9311 and designed with at least five replications and data points for all biological replicates are shown. Source data of Fig.5b, c, e, f, and h–oare provided as a Source Data file 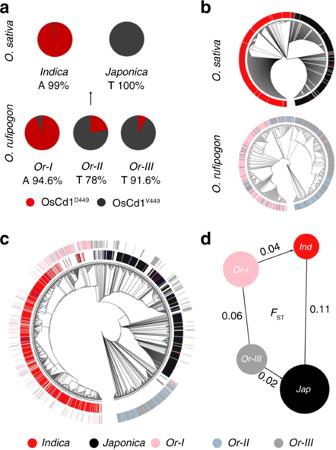Fig. 6 Genotypes and phylogenetic analysis ofOsCd1.aThe spectrum of allele frequencies at the causal polymorphisms ofOsCd1inO. rufipogon(Or-I, Or-II and Or-III) andO. sativa(japonicaandindica).bPhylogenetic tree of the full population calculated from the SNPs ofOsCd1inO. sativa(indicaandjaponicasubspecies, up) andO. rufipogon(Or-I, Or-II and Or-III, down).cPhylogenetic tree of the full population calculated from the SNPs ofOsCd1inO. rufipogon(outer ring) andO. sativa(inner ring).dIllustration of genetic diversity and population differentiation inO. rufipogonandO. sativa. TheFstvalues between the groups were indicated. ind,indica; jap,japonica. Or-I, Or-II and Or-III are colored in pink, light blue and gray respectively;indicaandjaponicasubspecies are in red and black, respectively The oligos used in constructing the sgRNA vectors for OsCd1 are listed in Supplementary Table 5 . The rice variety Nipponbare ( Oryza sativa L. ssp. japonica ) was used as the hosts in agrobacterium-mediated transformation for CRISPR-oscd1 mutant and ZH11 ( Oryza sativa L. ssp. japonica ) was used as the hosts in agrobacterium-mediated transformation for OE-OsCd1 lines (Hangzhou Biogle Co., LTD). The transgenic rice lines were grown in the paddy field in Hainan (18.48° N, 110.02° E, China), during normal rice-growing seasons. For CRISPR-oscd1 mutant lines, mature seeds were collected from T 0 plants and geminated for genotyping. Total DNA was isolated from transgenic plants and PCR was performed to amplify the genomic region surrounding the CRISPR target sites using the specific primers. The PCR fragments were directly sequenced by Sanger method to identify mutations. The CRISPR-oscd1 lines were then used for crossing with NIL and 9311 respectively and the T 1 plants was the functional complementary experiments. For the OE-OsCd1 lines, the GUS marker was used for the selection of pure rice lines in T 2 plants and then the pure rice lines were used for further experiments. Hydroponic experiments To conduct the hydroponic experiments in vegetative stage, rice seeds of wild-type rice and CRISPR-oscd1 lines were sown in a germination box with water in the dark. Then the 3-days rice were transferred to Kimura B solution containing (NH 4 ) 2 SO 4 , MgSO 4 ·7H 2 O, KNO 3 , Ca(NO 3 ) 2 ·4H 2 O, and KH 2 PO 4 and the micronutrients MnCl 2 ·4H 2 O, H 3 BO 3 , (NH 4 ) 6 Mo 7 O 24 ·4H 2 O, ZnSO 4 ·7H 2 O, CuSO 4 ·5H 2 O, and Fe-EDTA, pH 5.6. After growing in Kimura B solution 5 days, 1 μM CdCl 2 were added and the seedings were treated with CdCl 2 for 20 days. The plants were cultivated in the growth chamber at a temperature of 30 °C and the nutrient solution was replaced every 2 d. Then the shoot and root were collected separately with five replications to determine the Cd concentration. All the assays were performed at least three times. Pot and field experiments Pot experiments were carried out at the greenhouse of Institute of Botany, Beijing. Three-week seedlings of Nipponbare, CRISPR-oscd1 lines, 9311 and NILs pre-cultured hydroponically were transplanted to the pot with 0.18 mg kg −1 Cd in May and harvested at September. All experiments were repeated with 30 biological replicates. Field tests of 9311 and the NIL were performed during May to September in 2017 and 2018. All the cultivars were planted in the Cd-polluted paddy fields at Institute of Subtropical Agriculture, CAS. The soil Cd concentration was 1.80 mg kg −1 , pH 5.4. Randomized complete block design was applied in the field experiments. Each sample was assigned with three replicates. All the seedlings were transplanted at a spacing of 17 cm within rows and the distance between two rows was 20 cm. Following method was used to measure the agronomic traits including plant height, filled spikelet rate and grain yield per plant after harvest. Plant height was the length of main tiller; Filled spikelet rate was calculated as follows: filled grains/(unfilled grains + filled grains) × 100%; The grain yield was determined by weighing all the grains of one plant after drying at 50 °C in a lab oven for 8 h. The grain metal concentration was determined as described follows. Determination of metal accumulation using ICP-MS The content of total Cd, Zn, Mn, and Fe in the yeast and plant samples were determined by Inductive Coupled Plasma Emission Spectrometer (ICP-OES) (iCAP6300, Thermo Electron Corp., MA, USA). All samples were dried at 80 °C for 6 h. Dried samples were digested using 2 ml of concentrated HNO 3 overnight. Sample digestion was carried out by heating block at 200 °C for 8 h. After cooling, the digested solution was diluted to 15 ml with deionized water and filtered through 0.22 μm cellulose acetate membranes filters. All digestions were performed in triplicate. The blank HNO 3 was used as the negative control and the certified standard material sample (CRM rice; GBW100348) was used as the positive control. All the assays were performed at least three times. In situ analyses using synchrotron X-ray fluorescence Metal distribution in brown rice was evaluated using micro-X-ray fluorescence (SR- μXRF ) method, which performed at 4W1B beamline, Beijing synchrotron Radiation Facility. The longitudinal and latitudinal sections of rice samples were prepared for SR- μXRF analysis. The incident X-ray energy is 15 keV and the spot size diameter is 50 μm. Si (Li) solid state detector was used to detect X-ray fluorescence emission lines. Step-mode with 100*100 μm was used to acquire the two-dimensional mapping of rice grain samples and each step’s live time is 30 s. After sample mapping, the data processing was performed using PyMca package [63] and Origin 8. Quantitative real-time PCR Nipponbare varieties, 20 japonica and 20 indica cultivars were treated with and without 1 μM CdCl 2 for 24 h, respectively. Total RNA of the root, shoot and the whole plant was extracted using TRIzol reagent (Invitrogen) and then treated with DNase I. After DNaseI digest, ~2 μg RNA was converted to cDNA and the product was used as templates for the qPCR. Water and the cDNA without DNaseI digestion were used as negative control. qPCR was performed on an ABI 7500 instrument using SYBR Green PCR Master mix following the manufacturer's instructions (Takara, RR420). Oshiston gene were used as internal standards, and normalized relative expression was calculated by the ΔΔCt (cycle threshold) method. The primers used in qPCR are listed in Supplementary Table 4 . Tissue expression assay For histochemical analysis of GUS activity, the upstreaming 2.5 kb genomic fragment of OsCd1 was regarded as the OsCd1 promoter and cloned into pCAMBIA1391 to generate OsCd1 promoter ::GUS vector. The vectors were then transformed into Nipponbare and the transgenetic rice were sampled to detect GUS expression. To determine the activity of GUS, the samples were incubated into the solution containing 1 mM X - gluc, 10% methanol, 0.5% Triton X-100 and 50 mM Na 3 PO 4 at 37 °C for 24 h. After being stained, 75% ethanol was applied to remove chlorophyll. Resin semi-thin sections were prepared for image collection to determine GUS activity. For the GFP observation, the OsCd1 ’s promoter was cloned into pMDC45 and then the OsCd1 promoter ::GFP vector was then transformed into Nipponbare. The transgenetic rice root tissues were prepared into the frozen sections and then the confocal laser scanning microscope (FluoView FV1000, Olympus) was used to observe the location of OsCd1 . Nipponbare was used as the negative control and Ubi::GFP transgenetic rice was used as the positive control. Subcellular-localization assay The CDs of OsCd1 V449 and OsCd1 D449 were fused in frame with GFP via cloning into the binary vecor pMDC45. The resulting vectors pMDC45- OsCd1 V449 were transformed into Nipponbare ( Oryza sativa L. ssp. japonica ) and used as hosts in agrobacterium-mediated transformation method. For FM4-64 staining, rice root was transferred to 2.5 μM FM4-64 diluted in 1/2 MS medium for 3 min. Besides, the protoplasts were isolated from root and the pMDC45- OsCd1 V449 and pMDC45- OsCd1 D449 were transiently expressed in the root protoplasts for GFP observation. The subcellular localization and co-localization were evaluated using a confocal laser scanning microscope (FluoView FV1000, Olympus). Population genetics analysis 12 kb of the sequence centered on OsCd1 in 446 O. rufipogon accessions and 950 O. sativa varieties were obtained from rice HapMap3 data set ( http://server.ncgr.ac.cn/RiceHap3/ ). SNPs in the 12-kb region were used for the OsCd1 variety phylogenetic reconstruction analysis by MEGA7 using the neighbor-joining method with No. of differences model, pairwise deletion for missing data and 1000 bootstrap pseudoreplicates. Principal component analysis of the SNPs was performed using the software TASSEL. The level of population differentiation ( F st ) [64] and Tajima’s D [65] . Statistic was calculated by a custom PERL script using a 1000 bp window. The F st between Or-I and Or-III in O. rufipogon and between japonica and indica of O. sativa was calculated, respectively. NIL construction Oryza sativa near-isogenic line (NIL) were selected from a BC 5 F 2 , which was generated by crossing between japonica variety Nipponbare × indica variety 9311 then backcrossing to 9311, respectively. 120 SSR markers distributed evenly throughout 12 chromosomes were used for identification and selection of the candidate lines containing the target donor segment. The size of the introgression fragment in the NIL was about 1 Mb between RM3413 and RM3372. Reporting summary Further information on research design is available in the Nature Research Reporting Summary linked to this article.